Arginine clustering on calix[4]arene macrocycles for improved cell penetration and DNA delivery Cell-penetrating peptides are widely used as molecular transporters for the internalization inside cells of various cargo, including proteins and nucleic acids. A special role is played by arginine-rich peptides and oligoarginines covalently linked or simply mixed with the cargo. Here we report cell-penetrating agents in which arginine units are clustered on a macrocyclic scaffold. Instead of using long peptides, four single arginine units were covalently attached to either the upper or lower rim of a calix[4]arene, kept in the cone conformation building a ‘parallel’ cyclic array. These new macrocyclic carriers show high efficiency in DNA delivery and transfection in a variety of cell lines. Cell-penetrating peptides (CPPs) [1] , [2] , [3] are widely used as molecular transporters for the internalization of various molecular and macromolecular cargo inside cells. Among them, arginine-rich peptides, such as HIV-1 TAT fragments [3] , [4] and oligoarginines [5] , have a special role. They can be covalently linked to or, more simply, mixed with the cargo, both strategies showing examples of significant translocation activity [6] . Because of these features, arginine-rich peptides can also help the penetration of nucleic acids across the cell membranes opening interesting perspectives in gene delivery, which is a necessary prerequisite for gene therapy [7] , [8] , [9] , [10] , [11] . In this context, following a non-covalent approach [12] , [13] , CPPs are used in formulation, either simply with the nucleic acid filaments or in a ternary assembly, including also a cationic lipid. Alternatively, they can be covalently linked to a lipid structure ( Fig. 1a ) in which the resulting ratio between arginine units and lipophilic tails is, in general, of several to one [14] , [15] , [16] . A certain degree of rigidity imposed to the peptide structure, for example by cyclization of the arginine-rich sequences, seems to further enhance the cellular uptake [17] . We reasoned that the clustering of arginine units on a spatially well-defined macrocyclic scaffold ( Fig. 1b ) could be exploited to enhance their cell-penetrating properties, and we report here the first example of this strategy, applied to DNA delivery and cell transfection. Considering that cyclodextrins [18] and calixarenes [19] , [20] , [21] , [22] , [23] , [24] , [25] are non-toxic and have been used as scaffolds for building gene delivery systems, we selected calix[4]arene as the macrocyclic platform and anchored to it single arginine units rather than complex arginine-rich peptides, or linear and long oligoarginines, to limit to a ratio of one to one between amino acids and the lipophilic tails ( Fig. 1b ). Therefore, we herein describe the synthesis and the DNA binding and condensation properties of two new C-linked L -argininocalix[4]arenes and two acyclic Gemini-type analogues. Moreover, taking into account the several examples of polylysines used for cell transfection [26] , we also prepared a calixarene adorned at the upper rim with four L -lysine units, to verify the differences in activity related to the two types of amino acid. Gene-delivery studies with these compounds showed that the upper-rim arginine derivative 3a , in particular, has exceptional transfection properties and low cytotoxicity, suggesting that the proposed strategy of clustering arginine units on rigid, lipophilic macrocyclic scaffolds could be envisaged as a new approach to improve cell penetration of cargo. 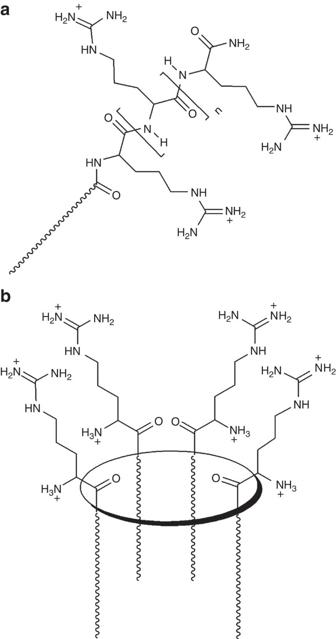Figure 1: Arginine arrays. (a) Linear versus (b) cyclic array. Ellipse represents a macrocyclic scaffold, wavy lines represent linear hydrocarbon chains. Figure 1: Arginine arrays. ( a ) Linear versus ( b ) cyclic array. Ellipse represents a macrocyclic scaffold, wavy lines represent linear hydrocarbon chains. Full size image Synthesis The upper rim tetraarginino- ( 3a ) and tetralysinocalix[4]arene ( 3b ), belonging to the class of C-linked peptidocalixarenes [27] , [28] , were prepared ( Fig. 2 ) starting from tetramino-tetrahexyloxycalix[4]arene 1 , selected on the basis of the previous experimental observation [19] , such that in the upper rim guanidinocalix[4]arene vectors the presence of hexyl chains at the lower rim allowed cell transfection in the absence of DOPE (1,2-dioleoyl-sn-glycero-3-phosphoethanolamine), with the same efficiency shown in the presence of this helper. The lower rim tetraargininocalix[4]arene 6 was synthesized from the tetrapropylamino precursor 4 ( [29] ; Fig. 2 ). In the synthetic pathway of both compounds 3a and 6 , by using N α -Boc- N ω -tosyl- L -arginine or N α -Fmoc- N ω -Mtr- L -arginine, the unexpected cleavage of the amide bonds between the amino acid units and the calixarene occurred during the deprotection steps. On the contrary, we did not observe this side reaction either when N α -Boc- N ω -Pbf- L -arginine (Boc- L -Arg(Pbf)-OH) and N α -Cbz- L- arginine were attached at the upper and at the lower rim of 1 and 4 , respectively, or during the removal of Boc groups from the lysine functionalized compound 2b . 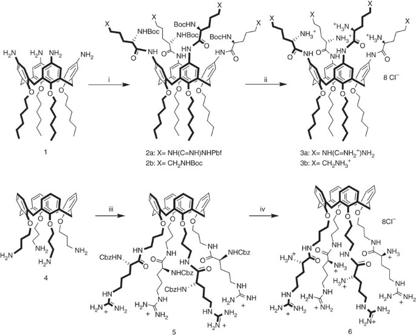Figure 2: Synthesis of peptidocalix[4]arenes 3a,b and 6. Reagents and conditions: (i) Boc-L-Arg(Pbf)-OH (Nα-Boc-Nω-Pbf-L-arginine),N-ethyl-N′-(3-dimethylaminopropyl)carbodiimide hydrochloride (EDAC), hydroxybenzotriazole (HOBt),N,N-dimethylaminopyridine (DMAP), dry CH2Cl2, rt, for2a, or Boc-L-Lys(Boc)-OH,O-(benzotriazol-1-yl)-N,N,N′,N′-tetramethyluronium hexafluorophosphate (HBTU), N,N-diisopropylethylamine (DIPEA), dry CH2Cl2, rt, for2b; (ii, 1) TFA/triisopropylsilane (TIS)/H2O (95/2.5/2.5), rt, for3a, or TFA/triethylsilane (TES)/CH2Cl2(10/2.5/87.5) at 0 °C for3b, (2) dil. HCl in methanol, pH 4, rt; (iii) Cbz-L-Arg-OH, N,N′-dicyclohexylcarbodiimide (DCC), HOBt, dry DMF, rt, SAX (strong anion exchange) sorbent (Cl−); (iv) H2/Pd(C), HCl, ethanol, rt. Boc:t-Butoxycarbonyl, Pbf: 2,2,4,6,7-pentamethyl-dihydrobenzofuran-5-sulfonyl, Cbz: carbobenzyloxy. Figure 2: Synthesis of peptidocalix[4]arenes 3a,b and 6. Reagents and conditions: (i) Boc- L -Arg(Pbf)-OH ( N α -Boc- N ω -Pbf- L -arginine), N -ethyl- N′ -(3-dimethylaminopropyl)carbodiimide hydrochloride (EDAC), hydroxybenzotriazole (HOBt), N,N -dimethylaminopyridine (DMAP), dry CH 2 Cl 2 , rt, for 2a , or Boc-L-Lys(Boc)-OH, O -(benzotriazol-1-yl)- N,N,N′,N′ -tetramethyluronium hexafluorophosphate (HBTU), N,N-diisopropylethylamine (DIPEA), dry CH 2 Cl 2 , rt, for 2b ; (ii, 1) TFA/triisopropylsilane (TIS)/H 2 O (95/2.5/2.5), rt, for 3a , or TFA/triethylsilane (TES)/CH 2 Cl 2 (10/2.5/87.5) at 0 °C for 3b , (2) dil. HCl in methanol, pH 4, rt; (iii) Cbz-L-Arg-OH, N,N′-dicyclohexylcarbodiimide (DCC), HOBt, dry DMF, rt, SAX (strong anion exchange) sorbent (Cl − ); (iv) H 2 /Pd(C), HCl, ethanol, rt. Boc: t- Butoxycarbonyl, Pbf: 2,2,4,6,7-pentamethyl-dihydrobenzofuran-5-sulfonyl, Cbz: carbobenzyloxy. Full size image The two Gemini-like derivatives ( 7 and 8 in Fig. 3 ) were prepared through similar procedures by successfully using Boc- L -Arg(Pbf)-OH for both (details in Supplementary Methods ). After standard deprotection reactions, the chloride salts of peptidocalixarenes 3a , b and 6 , and of non-macrocyclic compounds 7 and 8 were isolated. 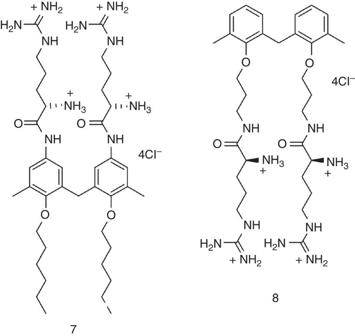Figure 3: Acyclic ligands. Gemini-type analogues of argininocalixarenes3aand6. For synthetic details relative to compounds7and8, and their precursors seeSupplementary Information. Figure 3: Acyclic ligands. Gemini-type analogues of argininocalixarenes 3a and 6 . For synthetic details relative to compounds 7 and 8 , and their precursors see Supplementary Information . Full size image All compounds resulted to be water soluble, but although 3a largely tends to form aggregates ( Supplementary Fig. S1 ) due to the presence of aliphatic chains at the lower rim, 6 showed sharp 1 H NMR signals in D 2 O ( Supplementary Fig. S2 ), ruling out self-assembly phenomena even in the presence of the high concentrations of the inorganic salts (NaCl and MgCl 2 ) added to the sample to increase the ionic strength and to reproduce more closely the conditions of the Atomic Force Microscopy (AFM) and transfection experiments. In the latter conditions, 3b , which is monomeric in pure D 2 O, self-assembles in species in slow exchange equilibrium on the NMR time scale with the monomer, whose signals progressively disappear by increasing the salt concentration ( Supplementary Fig. S3 ). This self-assembly activity, although not sufficient, seems an important prerequisite to induce DNA compactation and delivery. DNA binding and condensation Displacement of ethidium bromide ( Supplementary Fig. S4 ) and electrophoresis mobility shift assays ( Supplementary Fig. S5 ) evidenced the ability of all calixarene ( 3a , b and 6 ) and Gemini-like ( 7 and 8 ) conjugates to interact with plasmid EGFP-C1 (4731, bp) expressing for green fluorescent protein. AFM experiments in tapping mode on air allowed to visualize the different effects of each of them on the DNA folding ( Fig. 4 and Supplementary Fig. S6 ). The upper rim argininocalixarene 3a induces the DNA condensation to 50–60 nm globular species formed by a single ds -filament ( Fig. 4a ), and with proper dimension and compaction for cellular uptake. The lower rim arginino derivative 6 causes, on the contrary, the formation of large aggregates involving several filaments ( Fig. 4b ), partially reduced in size and in compaction degree by a decrease of the ligand concentration ( Supplementary Fig. S6a ). These multiplasmid aggregates are presumably too large to cross the cell membrane. Large aggregates are also formed by incubation of the plasmid with the lysino derivative 3b ( Supplementary Fig. S6b ), but the presence of DOPE, at a concentration double the calixarene, promotes the formation of small condensates ( Fig. 4c ) comparable in size with those obtained with 3a used alone. The treatment of DNA with the two non-macrocyclic compounds 7 and 8 , up to 10 μM concentration, does not generate globular condensates even if the interaction ability of the two ligands with the plasmids is unequivocally proved in AFM experiments by the DNA folding ( Supplementary Fig. S6c,d ), clearly different from the relaxed condition of the ds -filaments ( Fig. 4d ). 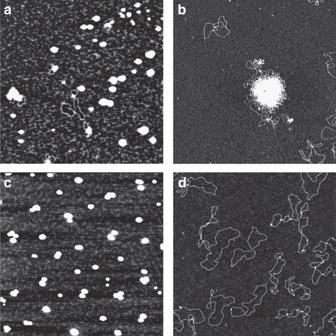Figure 4: AFM images of plasmid DNA. AFM images in tapping mode on air showing the effects induced on pEGFP-C1 plasmid DNA folding by incubation with (a) 2 μM argininocalixarene3a; (b) 1 μM argininocalixarene6; (c) 2 μM lysinocalixarene3bin presence of DOPE (1,2-dioleoyl-sn-glycero-3-phosphoethanolamine) 4 μM; and (d) image of pEGFP-C1 plasmid DNA 0.5 nM alone. Each image represents a 2 × 2 μm scan. Figure 4: AFM images of plasmid DNA. AFM images in tapping mode on air showing the effects induced on pEGFP-C1 plasmid DNA folding by incubation with ( a ) 2 μM argininocalixarene 3a ; ( b ) 1 μM argininocalixarene 6 ; ( c ) 2 μM lysinocalixarene 3b in presence of DOPE (1,2-dioleoyl-sn-glycero-3-phosphoethanolamine) 4 μM; and ( d ) image of pEGFP-C1 plasmid DNA 0.5 nM alone. Each image represents a 2 × 2 μm scan. Full size image Transfection properties To verify the ability of these compounds as gene-delivery systems, we selected for transfection the human Rhabdomyosarcoma (RD-4) cells because of their medical relevance and difficulty to be transfected by already established protocols and available formulations. A substantial agreement was found between the effect produced by the different ligands on the plasmid, observed by AFM ( Fig. 4 and Supplementary Fig. S6 ), and their ability and efficiency in the transfection process ( Fig. 5 and Supplementary Fig. S7 ). The argininocalixarene 6 resulted a very poor vector and only in the presence of the adjuvant DOPE was able to deliver pEGFP-C1 DNA (1 nM) in 5% of cells ( Fig. 5 and Supplementary Fig. S7 ). The failure of 6 as a gene-delivery system can be ascribed to the absence of a significant lipophilic region able to counterbalance the polarity of the substituents at the lower rim. Moreover, the shape of this ligand and the volume occupied by the polar heads with respect to the lipophilic portion constituted only by the aromatic cavity is apparently not suitable to induce aggregation phenomena able to support a transfection activity. Its Gemini-type analogue 8 failed in transfection also in the presence of the helper. On the contrary, the activity shown by the upper rim argininocalix[4]arene 3a is impressive. At 10 μM (cationic/anionic charges ratio N/P =8.4), it was able to transfect 75% of cells ( Fig. 5a ). Quite relevant is the comparison with its Gemini-type analogue 7 (9% of transfection but with DOPE) and with the commercially available LTX lipofectamine (35%) and polyethyleneimine (PEI; 41%) used as references ( Fig. 5b ). It is noteworthy the substantial inactivity observed for the lysine containing cluster 3b , whose efficiency is indeed boosted by DOPE to percentages of transfected cells (41%) only slightly lower than those obtained with the argininocalixarene 3a in presence of the adjuvant (46%). Particularly striking is that the highest transfection efficiency is reached by 3a without the helper lipid DOPE, which otherwise is usually exploited to enhance the vector efficiency and minimize its toxicity. This underlines the per se potency of this vector and, in the specific context of transfection, would allow, in perspective, the use of this macrocyclic cationic surfactant without helpers, thus simplifying the formulations. Remarkably, in the presence of serum the delivery properties of 3a are only slightly reduced with a transfection efficiency over 60%. 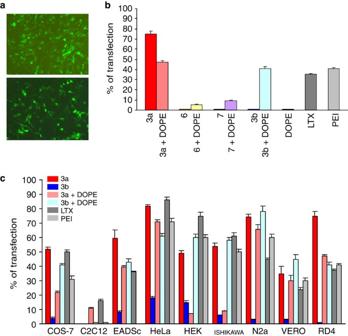Figure 5: Cell transfection experiments. (a) Images by fluorescence microscopy of human Rhabdomyosarcoma cells transfected (in green) upon treatment (at 48 h) with EGFP-C1 plasmid 1 nM formulated with (top) 10 μM calixarene3aand (bottom) LTX. In histogramb, transfection efficiency (at 48 h) to Rhabdomyosarcoma cells of argininocalix[4]arenes3aand6compared with the non-macrocyclic model7(20 μM), the lysinocalixarene3b, DOPE (1,2-dioleoyl-sn-glycero-3-phosphoethanolamine), LTX and PEI (polyethyleneimine). Error bars denote s.d. (n>3). In histogramc, transfection efficiency to other cell lines of argininocalixarene3a(red bar) compared with argininocalixarene3awith DOPE (pale red bar), lysinocalixarene3b(blue bar), lysinocalixarene3bwith DOPE (light blue bar), LTX (grey bar) and PEI (light grey bar). Calixarene derivatives and DOPE were used at 10 and 20 μM, respectively. Error bars denote s.d. (n>3). Figure 5: Cell transfection experiments. ( a ) Images by fluorescence microscopy of human Rhabdomyosarcoma cells transfected (in green) upon treatment (at 48 h) with EGFP-C1 plasmid 1 nM formulated with (top) 10 μM calixarene 3a and (bottom) LTX. In histogram b , transfection efficiency (at 48 h) to Rhabdomyosarcoma cells of argininocalix[4]arenes 3a and 6 compared with the non-macrocyclic model 7 (20 μM), the lysinocalixarene 3b , DOPE (1,2-dioleoyl-sn-glycero-3-phosphoethanolamine), LTX and PEI (polyethyleneimine). Error bars denote s.d. ( n >3). In histogram c , transfection efficiency to other cell lines of argininocalixarene 3a (red bar) compared with argininocalixarene 3a with DOPE (pale red bar), lysinocalixarene 3b (blue bar), lysinocalixarene 3b with DOPE (light blue bar), LTX (grey bar) and PEI (light grey bar). Calixarene derivatives and DOPE were used at 10 and 20 μM, respectively. Error bars denote s.d. ( n >3). Full size image The same results were substantially confirmed by experiments with luciferase ( Supplementary Fig. S8 ) again showing the higher efficiency of 3a with respect to the other ligands and LTX. The marked difference between the activity of 3a and that of its non-macrocyclic analogue 7 strengthens the hypothesis of a macrocyclic effect on the transfection process [21] . The rather low cytotoxicity of 3a ( Supplementary Fig. S9 ), which, quite unusually, increases in the presence of DOPE, is also worth noting. In particular, in transfection conditions the level of cell viability in the presence of this argininocalixarene ( Supplementary Fig. S9b ) is very close to that observed with LTX. The comparison between the structurally similar arginino cluster 3a and lysino-cluster 3b was widened by testing their transfection efficiency to other cell lines ( Fig. 5c ). Besides the C2C12 line to which both ligands resulted inactive and the LTX and PEI also have a very poor efficiency, in all other cases the superiority of the argininocalixarene 3a over the lysino analogue 3b , in absence of DOPE, appeared unequivocal ( Fig. 5c ). In fact for 3b , at the best 18% of transfected cells was observed in the case of Hela, while for 3a more than 80% of transfection was obtained in the treatment of this cell line, more than 70% with N2a, 60% with equine adipose-derived stromal cells (EADSCs), and more than 50% with Cos-7 and 40% with Vero cells. Moreover, excluding the cases of HEK cells, where LTX showed a significantly larger efficiency (75% versus ca. 50%), and of the above mentioned C2C12 cells, argininocalixarene 3a always resulted in a higher or at least comparable transfection activity with those of the references LTX and PEI. With EADSCs cell line, for instance, PEI was completely inefficient, whereas the 60% of transfection was obtained upon treatment with 3a that also almost doubled the LTX (36%). As in the experiments with RD-4 cells, the presence of DOPE, in general, decreased the transfection efficiency of 3a , drastically in some cases (COS-7, HEK, ISHIKAWA lines), even if a small activity with C2C12 cells was determined, which were not transfected at all in absence of adjuvant. On the other hand, the presence of DOPE transformed lysinocalixarene 3b in a vector ( Fig. 5c ), which was able to efficiently surpass the arginine cluster 3a in the case of HEK, ISHIKAWA, N2a and Vero cells, resulting in a better transfection efficiency for the latter two cell lines than all the other formulations. This further supports the idea that simple clustering on the cone calix[4]arene scaffold of a single unit of basic amino acid for lipophilic tail can effectively represent a novel winning strategy to build potent cell-penetrating systems. In conclusion, the clustering of only four units of basic amino acids, such as arginine and lysine, on a rigid macrocyclic scaffold like cone calix[4]arene, displaying two spatially well-defined regions, one apolar at the lower rim and one polar at the upper rim, gives rise to new, potent non-viral vectors for cell transfection. In particular, in the case of the tetraargininocalix[4]arene 3a , the one to one ratio between amino acid units and lipophilic tails is enough to reach this result, indicating that the circular array provided in this ensemble remarkably boosts the cell penetrating properties that arginine usually shows in linear oligomeric sequences and arginine-rich peptides, such as TAT HIV-1 fragments. The clearly higher efficiency of the arginino cluster 3a compared with analogue 3b bearing four lysine units, in absence of any adjuvant, underlines the superiority of arginine [30] and then of guanidinium group in conferring to the vector its cell penetrating properties. Moreover, the high transfection efficiency shown by the tetralysinocalix[4]arene 3b when used with DOPE confirms the efficacy of this clustering strategy. The novel amino acid arrangement present in the peptidocalix[4]arenes 3a and 3b also makes additional primary amino groups available, which might favour the protection of the vector–DNA complex from the lysosomal degradation and facilitate the release of DNA from the endosomes inside the cytosol, through the proton sponge effect [31] , [32] , [33] , [34] , and thus increasing the transfection efficiency of the vectors. All these features make argininocalix[4]arene 3a the progenitor of a new class of synthetic cationic surfactants, which could constitute a valuable alternative to commercially available formulations in transfection protocols, and suggest an unprecedented approach for the presentation of arginines in designing novel efficient cell-penetrating agents. General Moisture-sensitive reactions were carried out under a nitrogen atmosphere. Dry solvents were prepared according to standard procedures and stored over molecular sieves. Melting points were determined on an Electrothermal apparatus in capillaries sealed under nitrogen. 1 H and 13 C NMR spectra were recorded on Bruker AC300, AV300 and AV400 spectrometers (partially deuterated solvents were used as internal standards). For 1 H NMR spectra recorded in D 2 O at values higher than the room temperature, the correction of chemical shifts was performed using the equation δ =5.060−0.0122 × T (°C)+(2.11 × 10 −5 ) × T2 (°C), to determine the resonance frequency of water protons [35] . Electrospray ionization–mass spectrometry (ESI–MS) spectra were recorded on a single quadrupole instrument SQ Detector, Waters (capillary voltage 3.0–3.8 kV, cone voltage 30–160 eV, extractor voltage 3 eV, source block temperature 80 °C, desolvation temperature 150 °C, cone and desolvation gas (N 2 ) flow rates 1.6 and 8 l min –1 , respectively). High-resolution mass spectrometry (HRMS) spectra were recorded on a LTQ Orbitrap XL instrument in ESI mode. Thin-layer chromatography was performed on Merck 60 F 254 silica gel and Merck silica gel 60 RP-18. Flash column chromatography was performed on 230–400 mesh Merck 60 silica gel. HPLC purifications were performed on a 1100 Series Liquid Chromatograph Agilent, using an LC Detector. Strong anion-exchange (Cl − ) cartridges were used. 5,11,17,23-Tetrakis( L -Arg-amino)-25,26,27,28-tetrakis( n -hexyloxy)calix[4]arene octa-hydrochloride ( 3a ) A solution of calix[4]arene 2a (80 mg, 2.8 × 10 −2 mmol) in trifluoroacetic acid (TFA)/triisopropylsilane/H 2 O (95/2.5/2.5, 5 ml) was stirred at room temperature. The progression of the reaction was followed by ESI–MS. After completion, the volatiles were removed under reduced pressure, the solid residue repeatedly suspended in ethyl acetate (3 × 5 ml), and the organic solvent evaporated to help in removing the exceeding TFA. The crude material was then washed with distilled diethyl ether (3 × 7 ml) and removed after sample centrifugation. The trifluoroacetate anion of the resulting TFA octa-salt was exchanged with chloride by dissolving the solid in a methanol solution of concentrated HCl (pH=3–4) followed by evaporation (4 × ). Compound 3 was obtained as white solid (37 mg, 2.1 × 10 −2 mmol, 75%); melting point (mp): 230 °C dec; 1 H NMR (300 MHz, CD 3 OD): δ 7.18 (s, 4 H), 6.87 (s, 4 H), 4.47 (d, J =12.9 Hz, 4 H), 4.06 (bs, 4 H), 3.90 (t, J =7.3 Hz, 8 H), 3.40–3.20 (m, 8 H), 3.16 (d, J =12.9 Hz, 4 H), 1.98 (bs, 16 H), 1.72 (bs, 8 H), 1.50–1.20 (m, 24 H), 0.94 (t, J =6.3 Hz, 12 H); 13 C NMR (75 MHz, CD 3 OD): δ 167.9, 158.9, 155.1, 136.6, 136.5, 133.2, 122.6, 122.1, 77, 54.8, 42.2, 33.7, 32.4, 31.8, 30.2, 27.6, 25.9, 24.3, 14.8 (see Supplementary Fig. S10 ); MS ( m/z ): [M+2 H–8HCl] 2+ calcd. for C 76 H 132 Cl 8 N 20 O 8 , 723.5; found, 723.7; HRMS ( m/z ): [M+2 H–8HCl] 2+ calcd. for C 76 H 132 Cl 8 N 20 O 8 , 723.5028; found, 723.5027. Synthesis of 5,11,17,23-Tetrakis( L -Lys-amino)-25,26,27,28-tetrakis( n -hexyloxy)calix[4]arene octahydrochloride ( 3b ) A solution of calix[4]arene 2b (11.5 mg, 5.4 × 10 −3 mmol) in CH 2 Cl 2 /TFA/ triethylsilane (87.5/10/2.5, 1 ml) was stirred at 0 °C. The progression of the reaction was followed using MS. After completion, the volatiles were removed under reduced pressure. The crude material was suspended in diethyl ether (5 ml), centrifuged and the organic solvent removed (3 × ). The TFA anion of the resulting TFA octa-salt was exchanged with chloride by dissolving the solid in a methanol solution of concentrated HCl (pH=3–4) followed by evaporation (3 × ). Compound 3b was obtained as white solid (8.5 mg, quantitative); mp: 215 °C dec; 1 H NMR (300 MHz, CD 3 OD): δ 7.21 (d, J =2.4 Hz, 4 H), 6.85 (d, J =2.4 Hz, 4 H), 4.47 (d, J =12.9 Hz, 4 H), 4.03 (t, J =6.6 Hz, 4 H), 3.92 (t, J =7.5 Hz, 8 H), 3.15 (d, J =12.9 Hz, 4 H), 2.97 (t, J =7.5 Hz, 8 H), 2.08–1.83 (m, 16 H), 1.82–1.65 (m, 8 H), 1.63–1.25 (m, 32 H), 0.95 (t, 12 H, J =6.7 Hz); 1 H NMR (300 MHz, D 2 O, c =1 mM): δ 7.30 (d, J =2.4 Hz, 4 H), 6.85 (d, J =2.4 Hz, 4 H), 4.47 (d, J =13.0 Hz, 4 H), 4.12–3.95 (m, 12 H), 3.35 (d, J =13 Hz, 4 H), 3.02 (t, J =7.8 Hz, 8 H), 2.12–1.86 (m, 16 H), 1.82–1.62 (m, 8 H), 1.61–1.23 (m, 32 H), 0.94 (t, J =6.9 Hz, 12 H); 13 C NMR (150 MHz, CD 3 OD): δ 167.9, 154.8, 136.3, 133, 122.3, 121.8, 76.8, 54.7, 40.4, 33.4, 32.2, 32.1, 31.5, 28.2, 27.3, 24.1, 23.1, 14.6 (see Supplementary Fig. S11 ); MS ( m/z ): [M+2 H–8HCl] 2+ calcd. for C 76 H 132 Cl 8 N 12 O 8 , 667.5; found, 667.6; HRMS ( m/z ): [M+3 H–8HCl] 3+ calcd. for C 76 H 132 Cl 8 N 12 O 8 , 445.3294; found, 445.3293. 25,26,27,28-Tetrakis[3-( L -Arg-amino)propoxy]calix[4]arene octa-hydrochloride ( 6 ) Calix[4]arene 5 (80 mg, 4.1 × 10 −2 mmol) was dissolved in MeOH (13 ml) and a catalytic amount of Pd/C (10%) was added. Hydrogenation for the Cbz group removal was carried out at 2 atm in a Parr reactor for 24 h. Progression of the reaction was followed by 1 H NMR and ESI–MS. The reaction was quenched by catalyst filtration and the solvent removed under reduced pressure. Crude was dissolved in 10 ml water, filtered on a nylon 0.45-μm filter and purified by HPLC (column: Jupiter 4 μm Proteo 90 A, C-12, 90A, 10 × 250 mm, elution conditions: eluent A, H 2 O+0.1% formic acid; eluent B, MeOH+0.1% formic acid; 100% A over 5 min, 100% A to 84/16 A/B over 5 min, 84/16 to 74/26 A/B over 20 min, at 4 ml min −1 ). The fractions containing the pure product were collected and evaporated under reduced pressure. The formiate anion of the resulting salt was exchanged by adding HCl 37% to a methanol solution (5 ml) of the solid residue till pH 3, followed by evaporation under reduced pressure (4 × ) and liophilization, to give 6 as white powder (41 mg, 2.7 × 10 −2 mmol, 65%); mp: 182–185 °C; 1 H NMR (400 MHz, CD 3 OD): δ 8.70 (bt, 4 H), 6.63 (d, J =6.6 Hz, 8 H), 6.57 (t, J =6.6 Hz, 4 H), 4.44 (d, J =13.4 Hz, 4 H), 4.08 (t, J =6.4 Hz, 4 H), 4.02 (t, J =6.4 Hz, 8 H), 3.52 (t, J =6.8 Hz, 8 H), 3.30 (t, J =5.1 Hz, 8 H), 3.21 (d, J =13.4 Hz, 4 H), 2.33–2.12 (m, 8 H), 2.06–1.85 (m, 8 H), 1.81–1.63 (m, 8 H); 1 H NMR (300 MHz, D 2 O, c =2.4 mM): δ 6.84 (d, J =7.4 Hz, 8 H), 6.72 (t, J =7.4 Hz, 4 H), 4.41 (d, J =13.2 Hz, 4 H), 4.14–3.90 (m, 12 H), 3.72–3.55 (m, 4 H), 3.46–3.30 (m, 4 H), 3.35 (d, J =13.2 Hz, 4 H), 3.19 (t, J =6.9 Hz, 8 H), 2.36–2.10 (m, 8 H), 1.96–1.80 (m, 8 H), 1.70–1.52 (m, 8 H); 13 C NMR (100 MHz, CD 3 OD): δ 170.1, 158.6, 157.5, 136.1, 129.5, 123.4, 73.9, 54.1, 41.9, 38.4, 32, 31.2, 29.9, 25.6 (see Supplementary Fig. S12 ); MS ( m/z ): [M+2 H–8HCl] 2+ calcd. for C 64 H 108 Cl 8 N 20 O 8 , 639.4; found, 639.9; HRMS ( m/z ): [M+2 H–8HCl] 2+ calcd. for C 64 H 108 Cl 8 N 20 O 8 , 639.4089; found, 639.4087. The synthesis, characterization, spectroscopic information for all other compounds reported in the article and 1 H and 13 C NMR spectra ( Supplementary Figs S13 and S14 ) can be found in the Supplementary Methods . Cell culture and transient transfection assay RD-4 (human Rhabdomyosarcoma cell line (obtained from David Derse, National Cancer Institute, Frederick, MD)), C2C12 (mouse myoblast; ATCC (#CRL-1772)), N2a (mouse neuroblastoma; ATCC (#CCL-131)), EADSCs primary culture was obtained as described in Donofrio et al . [36] ), COS-7 (African green monkey kidney cells; ATCC (#CRL-1651)), VERO (African green monkey kidney cells; ATCC (#CCL-81)), HEK 293 (human embryo kidney cells; ATCC (#CRL-1573)), ISHIKAWA (human endometrial cancer cells; ECACC (#99040201)) and HeLa (human cervix adenocarcinoma; ATCC (#CCL-2)) were grown in EMEM medium containing NEAA, 10% fetal bovine serum, 2 mM L -glutamine, 100 IU ml −1 penicillin and 100 μg ml −1 streptomycin. All cultures were incubated at 37 °C in a humidified atmosphere containing 5% CO 2 . Cells were subcultured to a fresh culture vessel when growth reached 70–90% confluence (that is, every 3–5 days) and incubated at 37 °C in a humidified atmosphere of 95% air and 5% CO 2 . Transfections were performed in 24-well plates, when cells were 80% confluent (~5 × 10 4 cells) on the day of transfection. Plasmid (2.5 μg) and different concentrations of ligands were added to 1 ml of serum-free medium (DMEM, 2 mM L -glutamine and 50 μg ml −1 ), mixed rapidly and incubated at room temperature for 20 min. When used, serum was added at this point to the transfection solution. Following the removal of the culture medium from the cells, 0.5 ml of transfection mixture were carefully added to every well. Lipoplex formulations with helper lipid were prepared adding a 2 mM ethanol solution of DOPE to plasmid–ligand mixture at 1/2 ligand/DOPE molar ratio, where ligand concentration was kept to 10 μM. These solutions administered to the cells were completely clear and homogeneus. LTX transfection reagent was used according to manufacturer’s protocol as a positive transfection control. The mixture and cells were incubated at 37 °C in a humidified atmosphere of 95% air and 5% CO 2 for 5 h. Finally, transfection mixture was removed and 1 ml of growth medium added to each transfected well and left to incubate for 72 h. Five fields were randomly selected from each well without viewing the cells (one in the centre and one for each quadrant of the well) and examined. The transfected cells were observed under fluorescence microscope for enhanced green fluorescent protein expression. Each experiment was done at least three times. Statistical differences between treatments were calculated with student’s t -test and multifactorial analysis of variance. How to cite this article: Bagnacani, V. et al . Arginine clustering on calix[4]arene macrocycles for improved cell penetration and DNA delivery. Nat. Commun. 4:1721 doi: 10.1038/ncomms2721 (2013).